Autophagy enhances NFκB activity in specific tissue macrophages by sequestering A20 to boost antifungal immunity Immune responses must be well restrained in a steady state to avoid excessive inflammation. However, such restraints are quickly removed to exert antimicrobial responses. Here we report a role of autophagy in an early host antifungal response by enhancing NFκB activity through A20 sequestration. Enhancement of NFκB activation is achieved by autophagic depletion of A20, an NFκB inhibitor, in F4/80 hi macrophages in the spleen, peritoneum and kidney. We show that p62, an autophagic adaptor protein, captures A20 to sequester it in the autophagosome. This allows the macrophages to release chemokines to recruit neutrophils. Indeed, mice lacking autophagy in myeloid cells show higher susceptibility to Candida albicans infection due to impairment in neutrophil recruitment. Thus, at least in the specific aforementioned tissues, autophagy appears to break A20-dependent suppression in F4/80 hi macrophages, which express abundant A20 and contribute to the initiation of efficient innate immune responses. Autophagy is a highly conserved cellular process in eukaryotes, and is induced by various pathogen-associated molecular patterns and cytokines to eliminate intracellular microbes through autophagosomal digestion in mammals [1] , [2] , [3] . Autophagy can unselectively eliminate cytoplasmic proteins and organelles, and contributes to amino-acid recycling within a cell. At the same time, selective degradation of particular proteins is mediated by autophagy adaptor proteins such as p62, also called sequestosome-1, which contributes to maintenance of cellular activity. Recent studies have shown that autophagy eliminates assembled inflammasomes in macrophages [4] and BCL10 to limit T-cell receptor signalling in T cells [5] , both resulting in downregulation of immune responses. Thus, autophagy is currently known to suppress immune responses to protect hosts from possible collateral damage caused by overly active immunity [6] . It is reported that dectin-1, a fungal cell wall component β-glucan receptor, triggers conversion of microtubule-associated protein 1 light chain 3 (LC3)-I to LC3-II (ref. 7 ), which is used to monitor autophagy. A recent report demonstrated a protective role of autophagy in Candida infection [8] , while others showed that autophagy is not critical for host protection against C. albicans [9] , [10] . Thus, the specific role(s) of autophagy during Candida infection may be considered controversial. Various cell types in the host immune system play a protective role against Candida infection. For example, neutrophils prevent fungal growth and invasion, particularly at the early stage of infection. Therefore, neutropenia is a major causal factor in disseminated candidiasis [11] , [12] . Neutrophils prevent Candida hyphal formation by phagocytosed conidia, although macrophages are destroyed by germinated hyphae of ingested Candida [13] . As a result, neutrophils are viewed as critical cells for the host’s protection against Candida infection. Because of their short life span (half-life of ~6 h in circulation [14] ), prompt recruitment of neutrophils from bone marrow (BM) is critical for host protection. On the other hand, tissue-resident macrophages are considered to be an important source of neutrophil chemoattractants; thus, deletion of tissue-resident macrophages results in the failure of neutrophil recruitment and neutrophil-dependent immune responses [15] , [16] , [17] . F4/80 hi macrophages are largely tissue-resident [18] , [19] , [20] , [21] , although it is possible that F4/80 hi macrophages from different organs have tissue-specific phenotypes. In contrast, as previously demonstrated with BM chimera mice, 95–100% of F4/80 lo macrophages in various organs are replaced by donor BM cells [20] . It is also known that, during infection, F4/80 lo monocytes/macrophages are recruited in the infected sites [22] , [23] , while the spleen has a number of monocytes even in naive mice. Distinct gene expression pattern between F4/80 lo and F4/80 hi macrophages [20] suggests different functions between the two populations. Currently, it is unknown which macrophage subset is the main producer of neutrophil chemoattractants in fungal infection. Host cells are equipped with various mechanisms that negatively regulate immune responses to avoid hyperinflammation and autoimmunity. For example, A20 acts as a pivotal NFκB suppressor under Toll-like receptors (TLRs), and tumour necrosis factor receptor (TNFR) [24] . A20 deficiency causes severe autoimmune inflammation by excessive NFκB activation [25] , [26] , [27] . However, such a negative regulatory system, if sustained, hampers host immune responses to act quickly on the clearance of pathogens. In order to solve this dilemma, immune suppression by A20 must be strictly controlled when infections occur. Therefore, timely downregulation of A20 is considered to be important during acute infections. Although NFκB is known to induce A20 expression [28] , the mechanism underlying the negative regulation of A20 is not clear. In the current study, we evaluate antifungal immunity in mice conditionally lacking autophagy-related protein-7 (ATG7), essential for autophagosome formation [29] and LC3-associated phagocytosis [30] , in myeloid cells. Our data demonstrate that autophagy downregulates A20 in F4/80 hi macrophages through p62-associated autophagic sequestration and that the resulting NFκB activation induces expression of chemokines at an early stage of Candida infection. On the basis of these results, we suggest a mechanism by which autophagy protects hosts by enhancing NFκB signalling in tissue-resident macrophages, which indeed play a sentinel role at the early stage of fungal infections. Lack of ATG7 attenuates host resistance against Candida To assess the impact of ATG7 on fungal immunity, we generated Atg7 fl/fl lysozyme M ( LysM ) cre/+ mice (denoted as ‘ Atg7 CKO mice’ hereafter), in which myeloid cells, such as macrophages, dendritic cells (DCs) and neutrophils, lack autophagy. We confirmed that Atg7 mRNA expression was abolished in peritoneal macrophages ( Supplementary Fig. 1 ). When the mice were intravenously injected with either 10 6 ( Fig. 1a,b ) or 2 × 10 5 ( Fig. 1c,d ) conidia of Candida , weights and the survival of Atg7 CKO mice were significantly reduced compared with control LysM cre/+ mice (denoted as ‘WT mice’ hereafter). Importantly, the significant difference in weight reduction was observed on day 1 or 2 ( Fig. 1b,d ). Therefore, the impact of autophagy in myeloid cells on host protection was apparent at a very early stage (24–48 h) of fungal infection. We next compared fungal burdens in WT and Atg7 CKO mice in the kidney and spleen on day 3. Fungal loads in both organs were significantly increased in Atg7 CKO mice ( Fig. 1e ), and the increased fungal load was also histologically identified in the kidney ( Fig. 1f ). 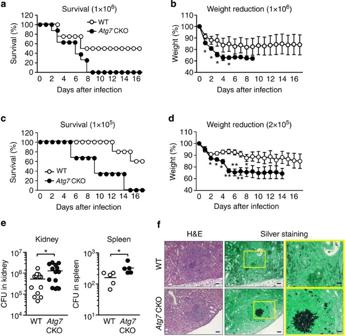Figure 1: Absence of ATG7 in myeloid cells decreases host resistance againstCandidainfection. (a–d)Atg7fl/flLysMcre/+(Atg7CKO) andLysMcre/+(WT) mice were systemically infected byi.v.injection ofC. albicans.Mouse survival (a,c) and weight (b,d) were monitored. Innocula ofCandidawere 106spores per mouse toAtg7CKO (n=9) and WT(n=12;a,b), and 2 × 105spores per mouse toAtg7CKO (n=12) and WT(n=10;c,d). (e) Fungal burdens in the kidney and the spleen ofAtg7CKO and WT mice 3 days after 106C. albicans i.v.injection. One circle denotes a result from one mouse. (f) Haematoxylin and eosine and silver staining of sections from kidneys of WT andAtg7CKO mice 3 days after 106C. albicans i.v.injection.Candidais observed with black in silver staining. Magnified views of the panels in the middle (yellow rectangles) are shown on the right. Scale bars in the left and middle panels indicate 200 μm; and scale bars in the panels on the right indicate 60 μm. Data are representative of independent two experiments. Error bars represent mean±s.d. Student’st-test was used for statistical analysis. *P<0.05, **P<0.01. Figure 1: Absence of ATG7 in myeloid cells decreases host resistance against Candida infection. ( a – d ) Atg7 fl/fl LysM cre/+ ( Atg7 CKO) and LysM cre/+ (WT) mice were systemically infected by i.v. injection of C. albicans. Mouse survival ( a , c ) and weight ( b , d ) were monitored. Innocula of Candida were 10 6 spores per mouse to Atg7 CKO ( n= 9) and WT (n= 12; a , b ), and 2 × 10 5 spores per mouse to Atg7 CKO ( n =12) and WT (n= 10; c , d ). ( e ) Fungal burdens in the kidney and the spleen of Atg7 CKO and WT mice 3 days after 10 6 C. albicans i.v. injection. One circle denotes a result from one mouse. ( f ) Haematoxylin and eosine and silver staining of sections from kidneys of WT and Atg7 CKO mice 3 days after 10 6 C. albicans i.v. injection. Candida is observed with black in silver staining. Magnified views of the panels in the middle (yellow rectangles) are shown on the right. Scale bars in the left and middle panels indicate 200 μm; and scale bars in the panels on the right indicate 60 μm. Data are representative of independent two experiments. Error bars represent mean±s.d. Student’s t -test was used for statistical analysis. * P< 0.05, ** P <0.01. Full size image ATG7 has no direct influence on fungal killing In an effort to describe the protection mechanism of autophagy in innate immune responses against fungal pathogen, we first examined whether or not Candida could induce autophagy in innate immune cells. Macrophage cell line (RAW-Blue cell) was cocultured with Candida conidia, and the induction of autophagy was evaluated by detecting LC3 puncta formation and LC3-II induction. Sixty minutes after the stimulation with conidia, LC3 puncta formation was clearly observed ( Fig. 2a ). Immunoblotting data also confirmed the induction of autophagy as quickly as 5 min following the coculture set-up ( Fig. 2b ). Autophagy is known to enhance phagocytosis of viral, bacterial and parasitic pathogens [1] , [2] , [3] . We thus next examined whether or not ATG7-mediated phagocytic activity in macrophages and neutrophils. The phagocytic capacity of both bone marrow-derived macrophages (BMDMs) and neutrophils, obtained from Atg7 CKO and WT mice, was assessed with flow cytometry. Unexpectedly, the absence of autophagy did not affect the percentages of host cells showing a fluorescent marker for Candida ( Fig. 2c,d ) and phagocytic index (the number of Candida detected with single macrophages; Fig. 2e ). No change in Atg7 CKO was found also in thioglycollate-elicited peritoneal and total splenic macrophages ( Supplementary Fig. 2 ). 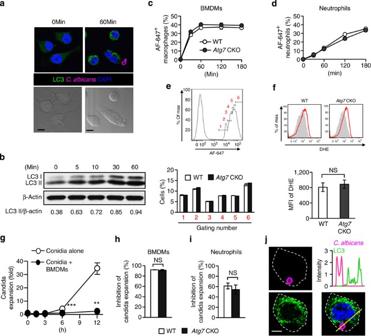Figure 2: Autophagy is induced byCandidabut does not play a role inCandidauptake by macrophages and neutrophils. (a) RAW-Blue cells (macrophage cell line) were cocultured withCandidalabelled with Alexa Fluor-647 (AF-647; pink) for 0 or 60 min at the 1:1 ratio of Raw-Blue and spore cells. LC3 and nuclei were shown with green and blue, respectively. Corresponding Nomarski images are shown below. Scale bars=5 μm. (b) Western blotting detection of LC3II in RAW-Blue cells stimulated withC. albicans(1:1 cell ratio) at the indicated time points. (c–e) BMDMs (c) and neutrophils (d) obtained fromAtg7CKO and WT mice were fluorescently labelled and cocultured with AF-647-labelledCandida(1:5 ratio of host cells andCandidaspores) for indicated duration. AF-647-positive cells were determined using flow cytometry. Intensity of AF-647 (Candida) in BMDMs at 30 min was assessed with flow cytometry analysis (e). The histogram is pre-gated on F4/80+. (f) To determine macrophage reactive oxygen species production, dihydroethidium (DHE) staining in BMDMs was evaluated using flow cytometry 2 h after coculture withCandida(1:1 ratio of BMDMs and spores). (g–i) Inhibition ofCandidaexpansion by BMDM (g,h) and neutrophils (i) was evaluated by the method described in the Methods section.Candidaexpansion with or without BMDMs was shown at indicated time points (g), and inhibition ofCandidaexpansion was evaluated at 12 h after coculture with host cell culture. (j) Intensity of LC3 signals (green) in aCandida(pink)-engulfed RAW-Blue cell at 60 min after starting coculture was analysed along with the yellow line in the panel at right bottom. Scale bar=2.5 μm. Shown ina,jare typical examples from 100 cells observed in four independent experiments. Results inb–iare representatives of at least two experiments with more than three mice per group. Error bars represent mean±s.d. Student’st-test was used for statistical analysis. NS; not significant. **P<0.01, ***P<0.001. Figure 2: Autophagy is induced by Candida but does not play a role in Candida uptake by macrophages and neutrophils. ( a ) RAW-Blue cells (macrophage cell line) were cocultured with Candida labelled with Alexa Fluor-647 (AF-647; pink) for 0 or 60 min at the 1:1 ratio of Raw-Blue and spore cells. LC3 and nuclei were shown with green and blue, respectively. Corresponding Nomarski images are shown below. Scale bars=5 μm. ( b ) Western blotting detection of LC3II in RAW-Blue cells stimulated with C. albicans (1:1 cell ratio) at the indicated time points. ( c – e ) BMDMs ( c ) and neutrophils ( d ) obtained from Atg7 CKO and WT mice were fluorescently labelled and cocultured with AF-647-labelled Candida (1:5 ratio of host cells and Candida spores) for indicated duration. AF-647-positive cells were determined using flow cytometry. Intensity of AF-647 ( Candida ) in BMDMs at 30 min was assessed with flow cytometry analysis ( e ). The histogram is pre-gated on F4/80 + . ( f ) To determine macrophage reactive oxygen species production, dihydroethidium (DHE) staining in BMDMs was evaluated using flow cytometry 2 h after coculture with Candida (1:1 ratio of BMDMs and spores). ( g – i ) Inhibition of Candida expansion by BMDM ( g , h ) and neutrophils ( i ) was evaluated by the method described in the Methods section. Candida expansion with or without BMDMs was shown at indicated time points ( g ), and inhibition of Candida expansion was evaluated at 12 h after coculture with host cell culture. ( j ) Intensity of LC3 signals (green) in a Candida (pink)-engulfed RAW-Blue cell at 60 min after starting coculture was analysed along with the yellow line in the panel at right bottom. Scale bar=2.5 μm. Shown in a , j are typical examples from 100 cells observed in four independent experiments. Results in b – i are representatives of at least two experiments with more than three mice per group. Error bars represent mean±s.d. Student’s t -test was used for statistical analysis. NS; not significant. ** P <0.01, *** P <0.001. Full size image Because flow cytometry does not distinguish Candida -engulfed host cells from those simply attaching to Candida , we eye-counted Candida -engulfed macrophages from at least 100 cells randomly captured with confocal microscopic images. The results also indicated that WT and Atg7 CKO macrophages had similar abilities to phagocytose Candida ( Supplementary Fig. 3 ). In addition, the generation of reactive oxygen species, toxic for ingested microbes including Candida , was also unaltered in Atg7 -deficient macrophages ( Fig. 2f ). Our ex vivo assay to evaluate host cell inhibition of Candida growth showed comparable results between WT and Atg7 CKO with BMDMs, thioglycollate-elicited peritoneal macrophages, total splenic macrophages and neutrophils ( Fig. 2g–i ; Supplementary Fig. 2b,d ). These results suggested that ATG7 likely does not play a role either in host cell-intrinsic functions to phagocytose, or in inhibiting expansion of Candida both in macrophages and neutrophils. This is in clear contrast to the role of autophagy in infections by viruses, bacteria and parasites. We then tried to evaluate the time course of live Candida engulfment in macrophages, particularly within LC3 cargos. A few conidia were phagocytosed at 5 and 10 min, and we could not evaluate the presence of Candida -containing LC3 cargos. Yet, complete phagocytosis of conidia was observed at 30, 45 and 60 min ( Supplementary Fig. 4a ). Unexpectedly, no conidia were found within LC3 cargos, but LC3 protein was rather randomly distributed ( Fig. 2j ; Supplementary Fig. 4a ; Supplementary Table 1 ). Spores contained within LC3 cargos were sought in at least 100 macrophages at each time point; however, we found no spores contained in LC3 cargos. As a positive control, we could confirm LC3 recruitment to zymosan particles ( Supplementary Fig. 4b,c ; Supplementary Table 1 ), as previously reported [7] . These data suggest that live Candida was not cleared in autophagosomes, and this is also a clear contrast to the role of autophagy against viruses, bacteria and parasites. Autophagy increases neutrophil recruitment Atg7 CKO mice showed severe weight reduction as early as day 1 ( Fig. 1b ). As neutrophils are responsible for Candida clearance at the early stage of infection [12] , [31] , we investigated whether the lack of autophagy affected neutrophil recruitment to the kidney and spleen at 4 and 24 h post infection (hpi). The 4-h time point was too early to statistically evaluate neutrophil infiltration; however, the result at 24 hpi using WT mice showed a sizeable increase in numbers of neutrophils ( Supplementary Fig. 5 ). At 24 hpi, the cellularity of total splenocytes in Atg7 CKO mice was comparable to that in WT mice ( Supplementary Fig. 6a ); however, Atg7 CKO mice showed significantly reduced neutrophil recruitment in both the kidney and spleen ( Fig. 3a,b ). Interestingly, WT mice showed a more drastic decrease in BM neutrophil population at 24 hpi than did Atg7 CKO mice after infection ( Fig. 3c ), while WT and Atg7 CKO naive mice had similar sizes of the BM neutrophil population in an uninfected condition ( Fig. 3d,e ). This suggests that Atg7 CKO mice had less neutrophil egress from the BM than did WT mice. To further evaluate the neutrophil recruitment to infected sites, we injected Candida to the peritoneal cavity of Atg7 CKO and WT mice. The lack of Atg7 significantly reduced recruitment of neutrophils in the peritoneal cavity ( Fig. 3f ). Collectively, these results suggest the general and noteworthy contribution of autophagy in neutrophil recruitment to inflammatory sites. 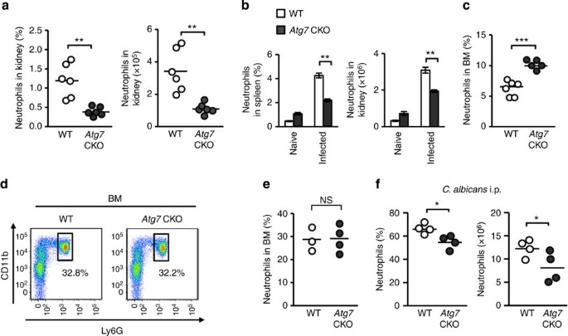Figure 3: Autophagy enhances neutrophil recruitment and clearance ofCandida. Indicated mouse groups receivedi.v.injection of 106Candidaspores (except forf), and neutrophils (CD11b+Ly6G+) were enumerated in indicated organs 24 h post infection using flow cytometry. (a,b) Proportions and numbers of neutrophils in the kidney from WT andAtg7CKO mice (a); moreover, in the spleen from naive or infected WT mice (b,n=4). (c–e) Proportions of neutrophils in BM 24 h afterCandidainfection (c). Representative flow cytometry CD11b/Ly6G-staining patterns (d) and proportions (e) of neutrophils in BM in naive mice. WT andAtg7CKO mice were compared. (f) Proportions and numbers of neutrophils infiltrated into the peritoneal cavity at 18 h afteri.p.injection of 5 × 106Candidaspores. One circle denotes a result from one mouse (a,e,f). Horizontal lines indicate the mean values. Data are representative of two independent experiments. Error bars represent mean±s.d. Student’st-test was used for statistical analysis fora,c,e,f) and analysis of variance (ANOVA) was used forb. NS; not significant. *P<0.05, **P<0.01, ***P<0.001. Figure 3: Autophagy enhances neutrophil recruitment and clearance of Candida. Indicated mouse groups received i.v. injection of 10 6 Candida spores (except for f ), and neutrophils (CD11b + Ly6G + ) were enumerated in indicated organs 24 h post infection using flow cytometry. ( a , b ) Proportions and numbers of neutrophils in the kidney from WT and Atg7 CKO mice ( a ); moreover, in the spleen from naive or infected WT mice ( b , n =4). ( c – e ) Proportions of neutrophils in BM 24 h after Candida infection ( c ). Representative flow cytometry CD11b/Ly6G-staining patterns ( d ) and proportions ( e ) of neutrophils in BM in naive mice. WT and Atg7 CKO mice were compared. ( f ) Proportions and numbers of neutrophils infiltrated into the peritoneal cavity at 18 h after i.p. injection of 5 × 10 6 Candida spores. One circle denotes a result from one mouse ( a , e , f ). Horizontal lines indicate the mean values. Data are representative of two independent experiments. Error bars represent mean±s.d. Student’s t -test was used for statistical analysis for a , c , e , f ) and analysis of variance (ANOVA) was used for b . NS; not significant. * P <0.05, ** P <0.01, *** P <0.001. Full size image We evaluated immune cells other than neutrophils in the spleen at 24 hpi. Proportions and numbers of splenic conventional DCs (cDCs) were slightly less in Atg7 CKO mice than in WT mice ( Supplementary Fig. 6b ), suggesting that recruitment of cDCs was somewhat affected by autophagy. Proportions and numbers of plasmacytoid DCs (pDCs), B cells, CD8 + and CD4 + T cells did not show a significant difference between WT and Atg7 CKO mice either before or after infection ( Supplementary Fig. 6c ). Numbers of F4/80 lo and F4/80 hi macrophage populations (gating strategy in Supplementary Fig. 6d ), were also unaltered ( Supplementary Fig. 6e ). In sum, increased numbers of neutrophils recruited to inflammatory sites appear to be important in autophagy-mediated host resistance during the early stage of Candida infection. Autophagy enhances production of neutrophil chemoattractants CXCR2 deficiency in mice reduces neutrophil influx into Candida -infected sites and increases susceptibility to gastric candidiasis and acute systemic candidiasis [32] . We first found that expression of CXCR2 was comparable between WT and Atg7 -deficient neutrophils in the BM, peripheral blood and the spleen ( Fig. 4a ). Chemotactic ability towards CXCL1 and CXCL2, CXCR2 ligands, was also comparable between WT and Atg7 -deficient neutrophils ( Fig. 4b ). These results suggested that Atg7 -deficient neutrophils have normal migration ability. We next assessed levels of major neutrophil chemoattractants in the serum and kidney at 24 hpi. Atg7 CKO mice showed significantly lower concentrations of both CXCL1 and/or CXCL2 in both the serum and kidney ( Fig. 4c,d ). These results suggest that autophagy increases neutrophil recruitment by enhancing production of chemoattractants at the site of inflammation, but not by enhancing the migratory ability of neutrophils. 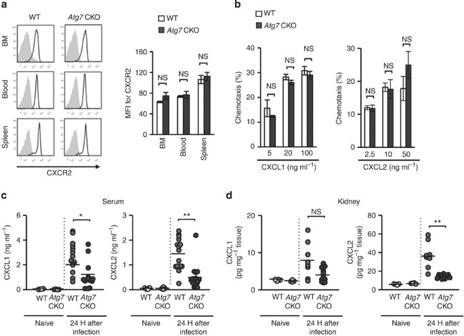Figure 4: Autophagy-induced levels of CXCL1 and CXCL2 in the serum and the kidney. (a) Histogram and mean fluorescent intensity (MFI) of CXCR2 staining determined with flow cytometry. Neutrophils were obtained from the BM, blood and spleen from WT andAtg7CKO mice at 24 h afteri.v.injection of 106Candidaspores. (b) Transwell migration assay of neutrophils towards CXCL1 and CXCL2. Neutrophils were FACS-sorted as CD11b+Ly6G+from the BM of naive mice and plated in the upper chamber of transwell. Indicated concentrations of CXCL1 and CXCL2 were added in the lower chamber. Cells were cultured for 1 h and the transmigration of neutrophils was assessed with flow cytometry. Data are representative of two independent experiments with at least three mice per each group (a,b). Error bars represent mean±s.d. (c,d) Levels of chemokines in the serum (c) and the kidney (d) from WT andAtg7CKO mice. Naive and infected mice at 24 h afteri.v.injection of 106Candidaspores were analysed. One circle denotes a result from one mouse. Horizontal lines indicate values of the mean. Error bars represent mean±s.d. ANOVA was used for statistical analysis ofa,band Student’st-test was used for (c,d). NS, not significant. *P<0.05, **P<0.01. Figure 4: Autophagy-induced levels of CXCL1 and CXCL2 in the serum and the kidney. ( a ) Histogram and mean fluorescent intensity (MFI) of CXCR2 staining determined with flow cytometry. Neutrophils were obtained from the BM, blood and spleen from WT and Atg7 CKO mice at 24 h after i.v. injection of 10 6 Candida spores. ( b ) Transwell migration assay of neutrophils towards CXCL1 and CXCL2. Neutrophils were FACS-sorted as CD11b + Ly6G + from the BM of naive mice and plated in the upper chamber of transwell. Indicated concentrations of CXCL1 and CXCL2 were added in the lower chamber. Cells were cultured for 1 h and the transmigration of neutrophils was assessed with flow cytometry. Data are representative of two independent experiments with at least three mice per each group ( a , b ). Error bars represent mean±s.d. ( c , d ) Levels of chemokines in the serum ( c ) and the kidney ( d ) from WT and Atg7 CKO mice. Naive and infected mice at 24 h after i.v. injection of 10 6 Candida spores were analysed. One circle denotes a result from one mouse. Horizontal lines indicate values of the mean. Error bars represent mean±s.d. ANOVA was used for statistical analysis of a , b and Student’s t -test was used for ( c , d ). NS, not significant. * P <0.05, ** P <0.01. Full size image Source of CXCL1 and CXCL2 early after C. albicans infection To determine the cellular source of CXCL1 and CXCL2, we sorted splenic F4/80 hi macrophages, F4/80 lo macrophages, cDCs, pDCs, natural killer cells, T cells and B cells, by fluorescence-activated cell sorting (FACS) from spleens of WT mice at 24 hpi, and then cultured the cells for 24 h. F4/80 hi macrophages were the only cell type that produced high levels of CXCL1 and CXCL2 ( Fig. 5a ). When F4/80 hi macrophages were depleted from total splenocytes, the levels were significantly reduced ( Fig. 5b ). Thus, F4/80 hi macrophages appear to be critical producers of CXCL1 and CXCL2. 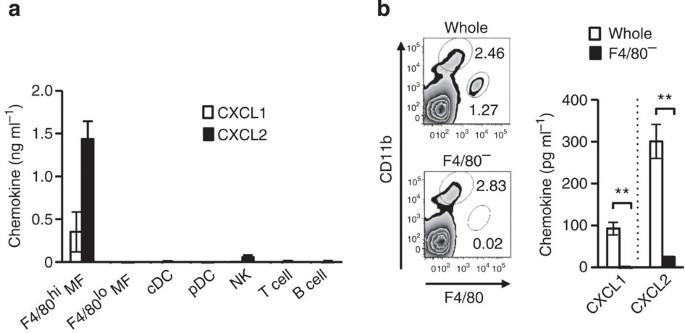Figure 5: F4/80himacrophages are a main source of CXCL1 and CXCL2 early afterCandidainfection. (a) CXCL1 and CXCL2 production by various splenic cell populations. Indicated splenic cell populations were purified using FACS from the spleen of mice 24 h after 106Candida i.v.inoculation, and each population was cultured for 24 h (106cells ml−1). The chemokine production in the supernatants was assessed with enzyme-linked immunosorbent assay (ELISA).n=3. (b) Splenocytes were obtained from mice 24 h afteri.v.injection of 106Candidaspores. F4/80himacrophage population was depleted by magnetic beads, and the rest of splenocytes were confirmed to be lacking the F4/80hipopulation with flow cytometry (left panels). Whole splenocytes and F4/80himacrophage-removed splenocytes (F4/80−) were cultured (5 × 107ml−1) for 24 h and chemokine production in the supernatants was evaluated with ELISA;n=3. Error bars represent mean±s.d. Student’st-test was used for statistical analysis. **P<0.01. Figure 5: F4/80 hi macrophages are a main source of CXCL1 and CXCL2 early after Candida infection. ( a ) CXCL1 and CXCL2 production by various splenic cell populations. Indicated splenic cell populations were purified using FACS from the spleen of mice 24 h after 10 6 Candida i.v. inoculation, and each population was cultured for 24 h (10 6 cells ml −1 ). The chemokine production in the supernatants was assessed with enzyme-linked immunosorbent assay (ELISA). n =3. ( b ) Splenocytes were obtained from mice 24 h after i.v. injection of 10 6 Candida spores. F4/80 hi macrophage population was depleted by magnetic beads, and the rest of splenocytes were confirmed to be lacking the F4/80 hi population with flow cytometry (left panels). Whole splenocytes and F4/80 hi macrophage-removed splenocytes (F4/80 − ) were cultured (5 × 10 7 ml −1 ) for 24 h and chemokine production in the supernatants was evaluated with ELISA; n =3. Error bars represent mean±s.d. Student’s t -test was used for statistical analysis. ** P <0.01. Full size image Autophagy enhances chemokine production We next examined the potential impact of Atg7 deficiency in the production of CXCL1 and CXCL2 in vivo . At 24 hpi, splenic WT F4/80 hi macrophages expressed significantly higher levels of Cxcl1 and Cxcl2 mRNA than did Atg7 -deficient F4/80 hi macrophages and F4/80 lo macrophages of WT and Atg7 −/− backgrounds ( Fig. 6a ). High levels of CXCL2 protein expression was also identified in splenic WT F4/80 hi macrophages, but not in Atg7 -deficient or F4/80 lo macrophages in infected mice ( Fig. 6b ). Similarly, gene expression of Ccl3 and Ccl4 was highly expressed in splenic WT F4/80 hi macrophages from infected mice ( Supplementary Fig. 7a ). (Note that CCL3 and CCL4 are ligands of C–C chemokine receptor 5, and act as chemoattractants for monocyte-derived macrophages and DCs [33] .) 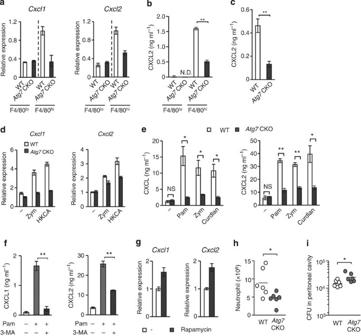Figure 6: ATG7 deficiency decreased chemokine production by F4/80hiperitoneal-resident macrophages (a) Levels ofCxcl1 and Cxcl2mRNA in splenic F4/80loand F4/80himacrophages obtained from WT andAtg7CKO mice 24 hpi with 106Candidaspores. (b) Levels of CXCL2 protein in supernatants of macrophages subsets indicated ina.n=3. (c) CXCL2 levels in culture supernatants of renal F4/80himacrophages from naive mice. Cells were stimulated with zymosan (100 μg ml−1) for 24 h.n=3. (d) Expression ofCxcl1andCxcl2mRNA in peritoneal F4/80himacrophages obtained from naive mice. Cells were stimulated with zymosan (Zym; 100 μg ml−1) or heat-killedCandida(HKCA; 5 × 105ml−1) for 3 h. (e) Levels of CXCL1 and CXCL2 proteins in culture supernatants of F4/80hiperitoneal macrophages stimulated with Pam3CSK4(Pam; 100 ng ml−1), zymosan (100 μg ml−1) or curdlan (100 μg ml−1) for 24 h.n=3. (f) Peritoneal F4/80himacrophages were pretreated with 3-MA (10 mM), and then stimulated 2 h later with Pam3CSK4(100 ng ml−1) for additional 24 h. Supernatants were analysed with ELISA to measure CXCL1 (left panel) and CXCL2 (right panel) production. (g) Peritoneal F4/80himacrophages were pretreated with rapamycin (1 μg ml−1) for 1 h, and then zymosan (100 μg ml−1) was added and harvested 3 h later.Cxcl1andCxcl2mRNA expression was assessed by real-time PCR analysis.n=3. (h,i) A million F4/80hiperitoneal macrophages of WT orAtg7CKO F4/80hiwere transferred into the peritoneal cavity ofAtg7CKO mice, and then 5 × 106Candidaspores werei.p.injected to the mice. Recruitment of neutrophils (h) and fungal burden (i) in the peritoneal cavity was evaluated 20 hpi. One circle denotes a result from one mouse. In all the experiments inFig. 6, except forh,i, cells were pooled from at least three mice for one group to get enough numbers of macrophages. Data are representative of at least two independent experiments. Error bars for mRNA data denote RQ-Max/Min as described in the Methods section. Error bars for protein data represent mean±s.d. ANOVA and Student’st-test were used fore,fandb,c, respectively. NS; not significantly different. *P<0.05 and **P<0.01. Figure 6: ATG7 deficiency decreased chemokine production by F4/80 hi peritoneal-resident macrophages ( a ) Levels of Cxcl1 and Cxcl2 mRNA in splenic F4/80 lo and F4/80 hi macrophages obtained from WT and Atg7 CKO mice 24 hpi with 10 6 Candida spores. ( b ) Levels of CXCL2 protein in supernatants of macrophages subsets indicated in a . n =3. ( c ) CXCL2 levels in culture supernatants of renal F4/80 hi macrophages from naive mice. Cells were stimulated with zymosan (100 μg ml −1 ) for 24 h. n =3. ( d ) Expression of Cxcl1 and Cxcl2 mRNA in peritoneal F4/80 hi macrophages obtained from naive mice. Cells were stimulated with zymosan (Zym; 100 μg ml −1 ) or heat-killed Candida (HKCA; 5 × 10 5 ml −1 ) for 3 h. ( e ) Levels of CXCL1 and CXCL2 proteins in culture supernatants of F4/80 hi peritoneal macrophages stimulated with Pam 3 CSK 4 (Pam; 100 ng ml −1 ), zymosan (100 μg ml −1 ) or curdlan (100 μg ml −1 ) for 24 h. n =3. ( f ) Peritoneal F4/80 hi macrophages were pretreated with 3-MA (10 mM), and then stimulated 2 h later with Pam 3 CSK 4 (100 ng ml −1 ) for additional 24 h. Supernatants were analysed with ELISA to measure CXCL1 (left panel) and CXCL2 (right panel) production. ( g ) Peritoneal F4/80 hi macrophages were pretreated with rapamycin (1 μg ml −1 ) for 1 h, and then zymosan (100 μg ml −1 ) was added and harvested 3 h later. Cxcl1 and Cxcl2 mRNA expression was assessed by real-time PCR analysis. n =3. ( h , i ) A million F4/80 hi peritoneal macrophages of WT or Atg7 CKO F4/80 hi were transferred into the peritoneal cavity of Atg7 CKO mice, and then 5 × 10 6 Candida spores were i.p. injected to the mice. Recruitment of neutrophils ( h ) and fungal burden ( i ) in the peritoneal cavity was evaluated 20 hpi. One circle denotes a result from one mouse. In all the experiments in Fig. 6 , except for h , i , cells were pooled from at least three mice for one group to get enough numbers of macrophages. Data are representative of at least two independent experiments. Error bars for mRNA data denote RQ-Max/Min as described in the Methods section. Error bars for protein data represent mean±s.d. ANOVA and Student’s t -test were used for e , f and b , c , respectively. NS; not significantly different. * P <0.05 and ** P< 0.01. Full size image We have shown that ATG7-sufficient splenic F4/80 hi macrophages produce high levels of chemokines both by in vivo and ex vivo. As Candida is accumulated in the kidney, we FACS-sorted renal F4/80 hi macrophages and stimulated the cells with zymosan ex vivo . Again, the absence of ATG7 in the cells reduced CXCL2 production ( Fig. 6c ). We next tested chemokine expression in F4/80 hi peritoneal macrophages, a dominant cell population in the peritoneal cavity of naive mice [21] . We obtained peritoneal-resident F4/80 hi macrophages, and then stimulated the cells ex vivo with either zymosan (a cell wall component from Saccharomyces cerevisiae ), heat-killed C. albicans (HKCA), Pam 3 CSK 4 or curdlan. Atg7 -deficient peritoneal F4/80 hi macrophages again showed reduced expression of CXCL1, CXCL2, CCL3 and CCL4 at the level of mRNA and/or protein after cell stimulation, compared with WT cells ( Fig. 6d,e ; Supplementary Fig. 7b ). As expected, WT peritoneal F4/80 hi macrophages expressed significantly higher levels of chemokines compared with WT peritoneal F4/80 lo ( Supplementary Fig. 8a ), as found in the splenic macrophages. The absence of ATG7 had no impact on CXCL2 production in F4/80 lo peritoneal macrophages ( Supplementary Fig. 8b ). Importantly, inhibition of autophagy with 3-methyladenine (3-MA) significantly reduced CXCL1 and CXCL2 production by WT F4/80 hi peritoneal macrophages stimulated with Pam 3 CSK 4 ( Fig. 6f ). Indeed, induction of autophagy by rapamycin treatment enhanced the gene expression of Cxcl1 and Cxcl2 induced by zymosan ( Fig. 6g ). As an additional representative of F4/80 lo macrophages, BMDMs were also tested. Atg7 -deficient BMDMs did not alter chemokine expression in CCL1, CCL2, CCL3 and CCL4 upon zymosan stimulation ( Supplementary Fig. 9a ). Further, treatment with rapamycin did not alter chemokine production by BMDMs ( Supplementary Fig. 9b ). Therefore, autophagy induces expression of tested chemokines in F4/80 hi macrophages but not in F4/80 lo macrophages. We then tested whether mice, intraperitoneally transferred with Atg7 -deficient F4/80 hi macrophages, have less ability to recruit neutrophils and clear Candida , compared with mice transferred with WT F4/80 hi macrophages. Less neutrophil recruitment and more fungal burden were identified in the peritoneal cavity of the recipients transferred with Atg7 -deficient F4/80 hi macrophages compared with those with WT F4/80 hi macrophages ( Fig. 6h,i ), although Atg7 deficiency in BMDMs transferred to the peritoneal cavity of recipients did not affect neutrophil recruitment and Candida clearance ( Supplementary Fig. 10 ). Taken together, results using various sources of macrophages suggested that ATG7 works through autophagy to induce chemokine production by F4/80 hi macrophages, and plays a critical role in neutrophil-mediated fungal clearance. Autophagy does not affect cell death or receptor expression We next sought to identify the mechanism for the autophagy-mediated induction of chemokine expression by F4/80 hi macrophages. First, there was no difference in cell survival between WT and Atg7 -deficient F4/80 hi macrophages ( Supplementary Fig. 11a ). Inhibition of autophagy with 3-MA in RAW-Blue cells also did not alter the proportion of live cells, compared with untreated cells ( Supplementary Fig. 11b ). Absence of autophagy did not seem to affect the expression levels of PRRs (pattern-recognition receptors) that detect Candida , such as TLR2, TLR4, dectin-1 and dectin-2, in F4/80 hi macrophages from the spleen, kidney and peritoneal cavity following Candida infection ( Supplementary Fig. 11c–e ). While F4/80 hi macrophages produce higher levels of chemokines than do F4/80 lo macrophages, this phenomenon was also not explained by expression levels of TLR2, TLR4, dectin-1 and dectin-2 ( Supplementary Fig. 12 ). These results suggested that autophagy contributes to enhancement of chemokine secretion in F4/80 hi macrophages without inhibiting cell death or upregulation of PRR expression. Here we have evaluated the ability of host cells to phagocytose Candida and to inhibit Candida growth, as shown in Fig. 2 and Supplementary Figs 2 and 3 , by using peritoneal F4/80 hi macrophages. Again, the absence of ATG7 in F4/80 hi macrophages did not alter Candida phagocytosis nor inhibited Candida growth, although LC3 puncta were clearly produced in WT F4/80 hi macrophages ( Supplementary Fig. 13a–d ). Interestingly, F4/80 hi macrophages were more susceptible than were F4/80 lo macrophages to intracellular germination of Candida ( Supplementary Fig. 13e–g ), suggesting that F4/80 hi macrophages are easily killed by Candida after completing their job as sentinels to recruit mainly neutrophils. Autophagy enhances NFκB activation in F4/80 hi macrophages A previous report showed that knockdown of either Atg5 or Atg7 inhibits NFκB signalling through TNFR [34] . Therefore, we sought to identify the mechanism in activation of NFκB, which induces gene expression of Cxcl1 , Cxcl2 , Ccl3 and Ccl4 (refs 35 , 36 , 37 ). We first confirmed that an NFκB inhibitor strongly suppressed CXCL1 and CXCL2 production by F4/80 hi peritoneal macrophages, stimulated with zymosan or HKCA ( Fig. 7a ). Indeed, Atg7 -deficient F4/80 hi macrophages showed lower levels of NFκB activity than did WT F4/80 hi macrophages, as demonstrated by less IκB phosphorylation, greater IκB levels (that is, less IκB degradation; Fig. 7b ), impaired NFκB p65 nuclear translocation ( Fig. 7c ; Supplementary Table 2 ) and impaired NFκB p65 binding to a target DNA promoter sequence ( Fig. 7d ). Inhibiting autophagy with 3-MA also downregulated NFκB activity in RAW-Blue cells detected with a secreted embryonic alkaline phosphatase (SEAP) reporter, and nuclear translocation assays ( Supplementary Fig. 14a ,b). Taken together, these results strongly suggest that autophagy positively regulates NFκB activation in F4/80 hi macrophages. 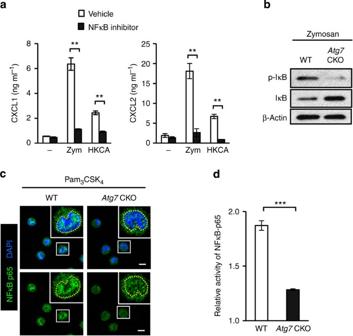Figure 7: Autophagy enhances NFκB activation in F4/80himacrophages. (a) Production of CXCL1 and CXCL2 by F4/80loand F4/80hiperitoneal macrophages. Cells were stimulated with zymosan (100 μg ml−1) or (HKCA; 5 × 105spores per ml) for 24 h with or without an NFκB inhibitor, QNZ. Culture supernatants were analysed with ELISA.n=3. (b) Western blot analysis of p-IκB and total IκB in F4/80hiperitoneal macrophages stimulated with zymosan (100 μg ml−1) for 30 min. (c) Translocation of NFκB p65 (green) to the nucleus (DAPI, blue) in F4/80hiperitoneal macrophages stimulated with Pam3CSK4(100 ng ml−1) for 30 min. NFκB localization was analysed with confocal microscopy. Yellow broken lines in enlarged photos indicate borders of the nucleus. Shown are representative images from at least 50 cells. Scale bars indicate 5 μm. (d) Relative activity of NFκB in WT andAtg7CKO F4/80hiperitoneal macrophages was evaluated. Cells were stimulated with zymosan (100 μg ml−1) for 30 min, and p62 binding to a target NF-κB response element in DNA was evaluated with colorimetric reading. Values were calculated as a fold increase of OD values of stimulated cells from those of unstimulated cells.n=3. Data are representative of two independent experiments. Error bars represent mean±s.d. ANOVA and Student’st-test were used for statistical analysis ofa,d, respectively. NS; not significant. ***P<0.001. Figure 7: Autophagy enhances NFκB activation in F4/80 hi macrophages. ( a ) Production of CXCL1 and CXCL2 by F4/80 lo and F4/80 hi peritoneal macrophages. Cells were stimulated with zymosan (100 μg ml −1 ) or (HKCA; 5 × 10 5 spores per ml) for 24 h with or without an NFκB inhibitor, QNZ. Culture supernatants were analysed with ELISA. n =3. ( b ) Western blot analysis of p-IκB and total IκB in F4/80 hi peritoneal macrophages stimulated with zymosan (100 μg ml −1 ) for 30 min. ( c ) Translocation of NFκB p65 (green) to the nucleus (DAPI, blue) in F4/80 hi peritoneal macrophages stimulated with Pam 3 CSK 4 (100 ng ml −1 ) for 30 min. NFκB localization was analysed with confocal microscopy. Yellow broken lines in enlarged photos indicate borders of the nucleus. Shown are representative images from at least 50 cells. Scale bars indicate 5 μm. ( d ) Relative activity of NFκB in WT and Atg7 CKO F4/80 hi peritoneal macrophages was evaluated. Cells were stimulated with zymosan (100 μg ml −1 ) for 30 min, and p62 binding to a target NF-κB response element in DNA was evaluated with colorimetric reading. Values were calculated as a fold increase of OD values of stimulated cells from those of unstimulated cells. n =3. Data are representative of two independent experiments. Error bars represent mean±s.d. ANOVA and Student’s t -test were used for statistical analysis of a , d , respectively. NS; not significant. *** P <0.001. Full size image Autophagy sequesters A20 to induce NFκB activation Since autophagy is known to specifically sequester certain proteins, we hypothesized that it also eliminates an NFκB signalling inhibitor to induce NFκB activity. For example, A20 is known to inhibit NFκB signalling [25] , [38] by deubiquitinating IκB kinase gamma (IKKγ; also known as NFκB essential modifier) and TRAF6 (ref. 39 ). A20-deficient mice spontaneously develop multiorgan inflammation and die prematurely [26] . Here we sought to show whether or not autophagy sequesters A20, particularly because A20 localize to an endocytic compartment upon stimulation with tumour necrosis factor (TNF)-α stimulation [40] . Stimulated Atg7 -deficient peritoneal F4/80 hi macrophages indeed showed higher levels of A20 protein than did WT F4/80 hi macrophages ( Fig. 8a ; Supplementary Fig. 15 ). Our time course results of A20 levels showed a peak at 1 h after Pam 3 CSK 4 stimulation for WT and Atg7 CKO macrophages; however, the initial increase in Atg7 -deficient F4/80 hi macrophages was much higher than that in WT cells ( Fig. 8a,b ). Even after the peak, Atg7 -deficient F4/80 hi cells maintained A20 levels significantly higher than those of WT F4/80 hi cells ( Fig. 8a,b ). As expected from previous studies [26] , the degree of NFκB activation showed a reverse correlation with A20 levels—weak NFκB activation in Atg7 CKO macrophages than WT macrophages ( Fig. 8a,b ). Here we confirmed highly K63-deubiquitinated IKKγ, suggesting the increased impact of A20 in Atg7 CKO F4/80 hi macrophages ( Fig. 8c ; negative controls in Supplementary Fig. 16a,b ). ATG7-specific downregulation of A20 did not occur at the mRNA level ( Fig. 8d ), suggesting post-translational downregulation of A20 in WT F4/80 hi macrophages. Indeed, autophagy negatively regulated A20 protein levels as evidenced by 3-MA treatment on WT F4/80 hi macrophage increasing A20 expression 1 h after Pam 3 CSK 4 stimulation ( Fig. 8e ). 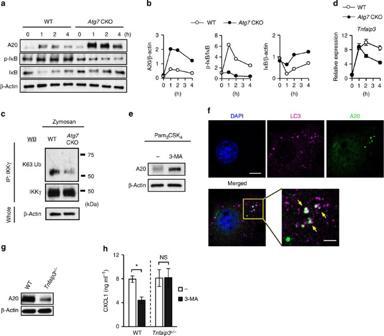Figure 8: Absence of ATG7 decreases A20 levels in F4/80himacrophages. (a,b) Turnover of A20, p-IκB and total IκB protein levels in F4/80hiperitoneal macrophages (WT versusAtg7CKO) stimulated with Pam3CSK4(100 ng ml−1). Cell lysates were harvested at indicated time points and submitted for western blot detection (a). Abundance of proteins evaluated by densitometry was plotted for A20, p-IκB normalized, total IκB normalized with β-actin, total IκB and β-actin, respectively. (c) Detection of K63-ubiquitination of IKKγ. F4/80hiperitoneal macrophages were stimulated with zymosan (100 μg ml−1) for 30 min. IKKγ was immunoprecipitated and K63-ubiquitination of IKKγ was detected by immunoblotting with K63-Ub antibody. Results of negative control using unstimulated cells and control IgG are shown inSupplementary Fig. 15a,b. (d) Expression ofTnfaip3mRNA in F4/80hiperitoneal macrophages (WT versusAtg7CKO) stimulated with Pam3CSK4(100 ng ml−1) for indicated duration. Evaluated by qPCR. Error bars for mRNA data denote RQ-Max/Min as described in the Methods section. (e) Expression of A20 in peritoneal F4/80himacrophages stimulated by Pam3CSK4(100 ng ml−1) for 1 h in the absence or presence of 3-MA (5 μM). (f) Confocal microscopy analysis to localize A20 and LC3. NIH-3T3 cells were transfected with V5-tagged A20 expression vector, and stimulated with Pam3CSK4(100 ng ml−1) for 60 min. LC3 and V5 antibodies were used to detect LC3 and A20, respectively. Scale bars in unmagnified and magnified panels indicate 10 and 4 μm, respectively. A20, LC3, and nuclei were shown with green, pink and blue, respectively. White arrows indicate colocalization of A20 and LC3. (g) Western blot detection of A20 in naive peritoneal F4/80himacrophages obtained from WT andTnfaip3+/−mice. (h) Levels of CXCL1 in culture supernatants of WT andTnfaip3+/−F4/80himacrophages stimulated with Pam3CSK4(100 ng ml−1) for 24 h. Indicated groups were treated with 3-MA (3 μM) starting an hour before the addition of Pam3CSK4. CXCL1 production was evaluated with ELISA.n=3. Data shown in all the panels are representatives of at least two independent experiments. Error bars represent mean±s.d. Student’st-test was used. NS; not significant. *P<0.05. Figure 8: Absence of ATG7 decreases A20 levels in F4/80 hi macrophages. ( a , b ) Turnover of A20, p-IκB and total IκB protein levels in F4/80 hi peritoneal macrophages (WT versus Atg7 CKO) stimulated with Pam 3 CSK 4 (100 ng ml −1 ). Cell lysates were harvested at indicated time points and submitted for western blot detection ( a ). Abundance of proteins evaluated by densitometry was plotted for A20, p-IκB normalized, total IκB normalized with β-actin, total IκB and β-actin, respectively. ( c ) Detection of K63-ubiquitination of IKKγ. F4/80 hi peritoneal macrophages were stimulated with zymosan (100 μg ml −1 ) for 30 min. IKKγ was immunoprecipitated and K63-ubiquitination of IKKγ was detected by immunoblotting with K63-Ub antibody. Results of negative control using unstimulated cells and control IgG are shown in Supplementary Fig. 15a,b . ( d ) Expression of Tnfaip3 mRNA in F4/80 hi peritoneal macrophages (WT versus Atg7 CKO) stimulated with Pam 3 CSK 4 (100 ng ml −1 ) for indicated duration. Evaluated by qPCR. Error bars for mRNA data denote RQ-Max/Min as described in the Methods section. ( e ) Expression of A20 in peritoneal F4/80 hi macrophages stimulated by Pam 3 CSK 4 (100 ng ml −1 ) for 1 h in the absence or presence of 3-MA (5 μM). ( f ) Confocal microscopy analysis to localize A20 and LC3. NIH-3T3 cells were transfected with V5-tagged A20 expression vector, and stimulated with Pam 3 CSK 4 (100 ng ml −1 ) for 60 min. LC3 and V5 antibodies were used to detect LC3 and A20, respectively. Scale bars in unmagnified and magnified panels indicate 10 and 4 μm, respectively. A20, LC3, and nuclei were shown with green, pink and blue, respectively. White arrows indicate colocalization of A20 and LC3. ( g ) Western blot detection of A20 in naive peritoneal F4/80 hi macrophages obtained from WT and Tnfaip3 +/ − mice. ( h ) Levels of CXCL1 in culture supernatants of WT and Tnfaip3 +/ − F4/80 hi macrophages stimulated with Pam 3 CSK 4 (100 ng ml −1 ) for 24 h. Indicated groups were treated with 3-MA (3 μM) starting an hour before the addition of Pam 3 CSK 4 . CXCL1 production was evaluated with ELISA. n =3. Data shown in all the panels are representatives of at least two independent experiments. Error bars represent mean±s.d. Student’s t -test was used. NS; not significant. * P <0.05. Full size image Here we hypothesized that autophagy sequesters A20, and sought to first identify LC3 and A20 colocalization. (In this regard, we had to overexpress A20 in 3T3 cells, since detection of endogenous A20 by confocal microscopy was difficult.). Although A20 was not colocalized with LC3 in unstimulated cells ( Supplementary Fig. 16c ), their colocalization was identified after cell stimulation ( Fig. 8f ; Supplementary Table 3 ). To further evaluate the impact of autophagy-mediated A20 downregulation in CXCL1 expression, we used Tnfaip3 +/ − (A20 heterozygous knockout) peritoneal F4/80 hi macrophages, which have reduced levels of A20 expression compared with WT macrophages ( Fig. 8g ). (Knocking down A20 and using Tnfaip3 homozygous knockout were not technically optional here, because of (1) poor ex vivo viability of F4/80 hi macrophages and (2) premature death in Tnfaip3 −/− mice by multiorgan inflammation [25] , [26] , respectively.) When autophagy was inhibited by 3-MA, CXCL1 production in WT cells was reduced, but no corresponding reduction was found in Tnfaip3 +/− cells ( Fig. 8h ), suggesting that autophagic removal of abundant A20 in WT cells played a role in high CXCL1 production. Impact of inhibiting autophagy in Tnfaip3 +/− macrophages was minimal due most likely to the fact that A20 was not sufficiently abundant in the Tnfaip3 +/− cells to make a difference with or without autophagy ( Fig. 8g ). In summary, these results strongly suggest that NFκB is activated by autophagic sequestration of A20 in F4/80 hi macrophages. p62 mediates the autophagic sequestration of A20 p62 is known as an adaptor protein that has a role in the selective delivery of target proteins to the autophagosome [41] . p62 was colocalized with A20 ( Fig.9a ; Supplementary Fig. 16d ; Supplementary Table 4 ) and co-immunoprecipitated with A20 ( Fig. 9b ; Supplementary Fig. 16e,f ) in naive and stimulated cells. These results strongly suggest an interaction between p62 and A20. In addition, a deficiency of Sqstm1 , encoding p62, increased protein levels of A20 in F4/80 hi macrophages ( Fig. 9c ; Supplementary Fig. 17a ), in which chemokine production was subsequently reduced ( Fig. 9d ; Supplementary Fig. 17b ). Collectively, it was thus suggested that p62 scavenges A20 to autophagic degradation and that the downregulation of A20 enhances NFκB activity for chemokine production. 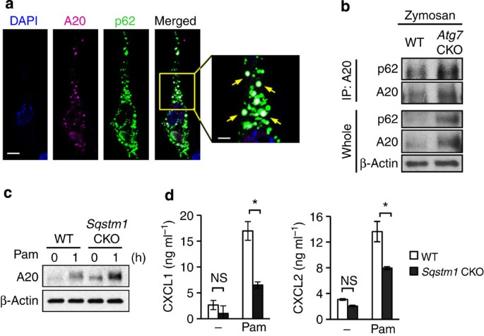Figure 9: p62 mediates A20 sequestration by autophagy. (a) Colocalization of A20 and p62 was evaluated with confocal microscopy. NIH-3T3 cells expressing exogenous A20-V5 and p62-HA were stimulated with Pam3CSK4(100 ng ml−1) for 60 min, and A20 (pink) and p62 (green) were detected by V5 and HA antibodies, respectively. Yellow arrows indicate co-localization of A20 and p62. Scale bar=10 μm. (b) Co-immunoprecipitation of A20 and p62. Peritoneal F4/80himacrophages were stimulated with Pam3CSK4(100 ng ml−1) for 60 min. Cell lysates were immunoprecipitated with A20 antibody, and then p62 was detected with p62 antibody by western blotting. Results for negative controls using unstimulated cells and control IgG are shown inSupplementary Fig. 15e,f. (c) Expression of A20 in WT and p62 (Sqstm1)-deficient peritoneal F4/80himacrophages, which were unstimulated or stimulated with Pam3CSK4(100 ng ml−1) for 1 h. (d) CXCL1 and CXCL2 production by WT and p62 (Sqstm1)-deficient peritoneal F4/80himacrophages. Macrophages were stimulated with Pam3CSK4(100 ng ml−1) for 24 h, and chemokine levels in the culture supernatants were evaluated by ELISA.n=3. Data in all the panels are representative of at least two independent experiments. Error bars represent mean±s.d. ANOVA was used for statistical analysis. NS; not significant. *P<0.05. Figure 9: p62 mediates A20 sequestration by autophagy. ( a ) Colocalization of A20 and p62 was evaluated with confocal microscopy. NIH-3T3 cells expressing exogenous A20-V5 and p62-HA were stimulated with Pam 3 CSK 4 (100 ng ml −1 ) for 60 min, and A20 (pink) and p62 (green) were detected by V5 and HA antibodies, respectively. Yellow arrows indicate co-localization of A20 and p62. Scale bar=10 μm. ( b ) Co-immunoprecipitation of A20 and p62. Peritoneal F4/80 hi macrophages were stimulated with Pam 3 CSK 4 (100 ng ml −1 ) for 60 min. Cell lysates were immunoprecipitated with A20 antibody, and then p62 was detected with p62 antibody by western blotting. Results for negative controls using unstimulated cells and control IgG are shown in Supplementary Fig. 15e,f . ( c ) Expression of A20 in WT and p62 ( Sqstm1 )-deficient peritoneal F4/80 hi macrophages, which were unstimulated or stimulated with Pam 3 CSK 4 (100 ng ml −1 ) for 1 h. ( d ) CXCL1 and CXCL2 production by WT and p62 ( Sqstm1 )-deficient peritoneal F4/80 hi macrophages. Macrophages were stimulated with Pam 3 CSK 4 (100 ng ml −1 ) for 24 h, and chemokine levels in the culture supernatants were evaluated by ELISA. n =3. Data in all the panels are representative of at least two independent experiments. Error bars represent mean±s.d. ANOVA was used for statistical analysis. NS; not significant. * P <0.05. Full size image F4/80 hi macrophages express high levels of A20 We then asked why the autophagy-mediated NFκB activation is specific for F4/80 hi macrophages. F4/80 hi macrophages expressed higher levels of Tnfaip3 (A20) mRNA than do F4/80 lo macrophages and BMDMs both with and without cell stimulation ( Fig. 10a ). Further, Western blotting showed high levels of A20 protein, particularly in Atg7 -deficient F4/80 hi macrophages after zymosan stimulation, while levels of A20 in F4/80 lo macrophages were too weak to be detected regardless of Atg7 deficiency ( Fig. 10b ). Even without stimulation, F4/80 hi macrophages expressed A20 protein abundant enough to be detected in by western blotting ( Supplementary Fig. 16e,f ). These results suggest that F4/80 hi macrophages express higher levels of A20 than do F4/80 lo macrophages regardless of cell stimulation. In addition, A20 and p62 appeared to constitutively interact ( Supplementary Fig. 16e ), suggesting that A20 is ready to be sequestered in autophagsomes with p62 as soon as autophagosomes appear. Sequestration of A20 in F4/80 hi macrophages by autophagy thus appears to be a critical event for robust NFκB activation upon fungal infection. Deficiency of autophagy allows accumulation of A20 in F4/80 hi macrophages, presumably contributing to the defect in their chemokine expression. Our results here suggest that tissue-resident F4/80 hi macrophages take advantage of autophagy to sequester intrinsically abundant A20 for the activation of NFκB in an effort to quickly respond to fungal infection ( Fig. 10c ). 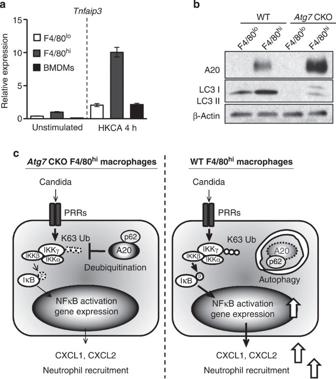Figure 10: A20 is highly expressed in F4/80hiperitoneal macrophages, but not in F4/80loperitoneal macrophages. (a) Comparison ofTnfaip3mRNA levels among F4/80loand F4/80hiperitoneal macrophages and BMDMs. Unstimulated and stimulated cells with HKCA (5 × 105ml−1, 1:1 ratio) for 4 h were analysed with real-time PCR. Error bars denote RQ-Max/Min as described in the Methods section. (b) Western blot analysis of A20 and LC3 expression in F4/80loand F4/80hiperitoneal macrophages stimulated with zymosan (100 μg ml−1) for 30 min. Data are representative of two independent experiments (a,b). (c) Schematic illustration of autophagy-mediated NFκB activation in F4/80himacrophages and the resulting induction of resistance toCandidainfection. F4/80himacrophages induce autophagy uponCandidadetection. Autophagy then sequesters abundant A20 through interaction between p62 and A20, and then unleashes NFκB activity in F4/80himacrophages. As a result, the macrophages secrete high levels of CXCL1 and CXCL2 to recruit neutrophils for fungal clearance. Figure 10: A20 is highly expressed in F4/80 hi peritoneal macrophages, but not in F4/80 lo peritoneal macrophages. ( a ) Comparison of Tnfaip3 mRNA levels among F4/80 lo and F4/80 hi peritoneal macrophages and BMDMs. Unstimulated and stimulated cells with HKCA (5 × 10 5 ml −1 , 1:1 ratio) for 4 h were analysed with real-time PCR. Error bars denote RQ-Max/Min as described in the Methods section. ( b ) Western blot analysis of A20 and LC3 expression in F4/80 lo and F4/80 hi peritoneal macrophages stimulated with zymosan (100 μg ml −1 ) for 30 min. Data are representative of two independent experiments ( a , b ). ( c ) Schematic illustration of autophagy-mediated NFκB activation in F4/80 hi macrophages and the resulting induction of resistance to Candida infection. F4/80 hi macrophages induce autophagy upon Candida detection. Autophagy then sequesters abundant A20 through interaction between p62 and A20, and then unleashes NFκB activity in F4/80 hi macrophages. As a result, the macrophages secrete high levels of CXCL1 and CXCL2 to recruit neutrophils for fungal clearance. Full size image In viral, bacterial and parasitic infections, autophagy contributes to host protection by containing pathogens in the autophagosome for pathogen clearance [1] , [2] , [3] . Autophagy also promotes phagocytosis and antigen processing in these microbial infections [42] , [43] , [44] . On the basis of these findings, we initially expected the involvement of autophagy in the direct killing of fungal pathogens. However, the data in this study demonstrated that ATG7 did not affect Candida phagocytosis or the inhibition of Candida expansion by macrophages and neutrophils. Unexpectedly, our intensive search did not identify LC3 cargos containing live Candida spores, although zymosan particles successfully recruited LC3. In line with our findings, an in vivo study using zebrafish also demonstrated that very few conidia of C. albicans were contained in LC3 cargos [45] . In addition, a recent study showed that live Candida did not induce clear LC3 staining surrounding conidia, while HKCA and β-1,3-glucan-coated polystyrene beads were clearly engulfed by LC cargos [46] , suggesting that live Candida somehow escapes from uptake by LC3 cargos. Although the possibility of transient inclusion of live Candida in LC3 cargos has not been ruled out, host cells do not appear to directly kill Candida in autophagosomes and LC3-associated phagosomes. A recent article reported that disruption of host autophagy ex vivo by Atg5 shRNA in a macrophage cell line decreased the phagocytic index of Candida , as well as the level of Candida -killing activity [8] . This result is not quite the same as what we found here; however, multiple differences exist between the earlier study’s experimental conditions and ours, as follows: the study [8] used the SC5314 Candida strain, Atg5 knockdown in J774.16 cell lines, and evaluated phagocytosis and Candida -killing activity at 30 min. On the other hand, we used Atg7 CKO in BMDMs, splenic macrophages, thioglycollate-elicited peritoneal macrophages and neutrophils ( Fig. 2c–e ; Supplementary Figs 2 and 3 ). We also evaluated phagocytosis at 0.5, 1, 2 and 3 h, as well as the inhibition of Candida expansion at 1.5, 3, 6 and 12 h. Despite these differences, a key conclusion of our study is the same as the previous report [8] in terms of the involvement of autophagy in host protection against Candida . We should also note another recent research effort that found only slightly worse survival from Candida infection in Atg7 CKO (LysM-Cre) mice [9] . One possible explanation of the latter is that the recent study [9] used another different Candida strain, because Candida strains are indeed known to have a significant impact on host responses [47] , [48] . Here we demonstrated autophagy-mediated induction of chemokine expression by sequestering an NFκB inhibitor, A20, in a manner specific to the F4/80 hi macrophage population at the least in spleens, the peritoneal cavity and the kidney during systemic Candida infection. A20 is also known to act as a negative regulator of autophagy [49] , suggesting that fine-tuning of inflammatory responses by feedback between A20 and autophagy is also possible in F4/80 hi tissue-resident macrophages. A20 works in TLR and TNFR signalling pathways, and protects hosts from collateral damage due to excessive inflammation initiated by viral and bacterial infections [25] , [26] , [27] , [50] . However, the role of A20 in fungal infection has not yet been reported. Here we suggest that abundant A20 in F4/80 hi macrophages is an obstacle to jump-start early innate immune responses in fungal infections. Thus, F4/80 hi macrophages are able to take advantage of autophagy and remove A20, since the cell type already has high levels of A20. The removal of A20 by autophagy in F4/80 hi macrophages subsequent to infection is thus an effective approach to address infection, and prepare for the next step, that is, recruitment of neutrophils. Given that Atg7 CKO mice are susceptible to Candida infection at an early stage, autophagy in F4/80 hi macrophages appears to be a critical and effective intervention, particularly at these earlier stages. A previous report demonstrated that autophagy eliminates BCL10, and inhibits NFκB activity in T cells upon T-cell receptor stimulation [5] . On the other hand, our results clearly indicate that autophagy enhances NFκB signalling by eliminating A20 in F4/80 hi macrophages. Since BCL10 is also expressed in macrophages, it is possible that BCL10 is also sequestered by autophagy in macrophages upon PRR stimulation; however, the autophagy-mediated depletion of BCL10 in macrophages may not have the impact it does in T cells, because signalling pathways inhibited by A20 have a significant impact on responses of macrophages. It is therefore likely that outcomes of autophagy are not the same between different cell types because of their distinct signal transduction networks. We have shown that autophagy removes abundant A20 in F4/80 hi macrophages for copious production of CXCL1/2. Here F4/80 lo macrophages also perform autophagy and do not express abundant A20 as F4/80 hi macrophages do. Nevertheless, F4/80 lo macrophages express low levels of CXCL1/2. Although further investigation is necessary to better explain why F4/80 lo macrophages do not produce CXCL1/2 as well as F4/80 hi macrophages, mechanistic machineries to produce the chemokines between the subsets appear to differ. For example, it is possible that expression of Cxcl1 and Cxcl2 genes in F4/80 lo macrophages may require a higher threshold of PRR signalling intensity than that in F4/80 hi macrophages. A possible impact of negative regulators on chemokine expression, other than A20 in F4/80 lo macrophages, cannot be ruled out as well. At the least, the ability to express high levels of CXCL1/2 by F4/80 hi macrophages as tissue-resident sentinels in the kidney, spleen and peritoneum is biologically relevant for early antifungal immunity; moreover, F4/80 hi macrophages may have further developed a mechanism for quickly secreting high levels of chemokines during the course of evolution. Hosts are protected from hyperinflammation and autoimmunity by the inhibitory effect of A20. At the same time, A20 becomes an obstruction when activation of immune responses is necessary during infections. For exerting rapid and strong immune responses, autophagy quickly sequesters inhibitory molecule A20, which is bound by p62 even before cell stimulation, in F4/80 hi macrophages for them to enhance NFκB activation for producing neutrophil chemoattractant ( Fig. 10c ). Autophagy plays a crucial role in early antifungal immunity by jump-starting the innate immune system in F4/80 hi macrophages, which are largely tissue-resident macrophages [18] , [19] , [20] , [21] . It would be helpful if future research efforts focus on whether or not targeted manipulation limited to tissue-resident macrophages is possible. This would allow researchers to further dissect the biology of tissue-resident macrophages in vivo . Results from the current study suggest that F4/80 hi macrophages do, indeed, play the role of a sentinel of immunity at the front lines of infection by utilizing autophagy. Mice and cell preparation All the mice used here are on the C57BL/6 background. Atg7 fl/fl , Tnfaip3 −/− and Sqstm1 fl/fl mice were described previously [51] , [52] , [53] . LysM cre/cre mice were purchased from Jackson Laboratories. Six- to eight-week-old sex-matched WT, Atg7 CKO, Tnfaip3 +/− or Sqstm1 CKO mice were used for all experiments. All the experiments were performed as approved by the Institutional Animal Care and Use Committee. Complete RPMI medium (10% (vol/vol) fetal bovine serum, penicillin/streptomycin (Sigma), 2 mM of L-glutamine; Life technologies)) was used for host cell culture. RAW-Blue cells were purchased from Invivogen. F4/80 hi and F4/80 lo macrophages were isolated from the kidney or peritoneal cavity using FACS isolation as CD11b + Ly6G − F4/80 hi and CD11b + Ly6G − F4/80 lo , respectively. Splenic F4/80 hi and F4/80 lo macrophages were isolated as AF + Ly6G − F4/80 hi and CD11b + Ly6G − F4/80 lo after gating out SSC hi (eosinophils). BMDMs were derived by culturing BM cells with L929 conditioned medium (15%, vol/vol) for 7 days as previously described [54] . Thioglycollate-elicited macrophages and neutrophils were obtained from the peritoneal cavity 3 days and 1 day, respectively, after intraperitoneal ( i.p. ) injection of thioglycollate (3%, 2.5 ml per mouse). For some experiments, thioglycollate-elicited macrophages and neutrophils were purified by MACS beads (Myltenyi) as CD11b + and Ly6G + cells, respectively. Total splenic CD11b + macrophages were purified from the spleen of naive mice with CD11c-MACS beads (Myltenyi). For chemotaxis assay, neutrophils were FACS-purified from BM of naive mice as CD11b + Ly6G + . On the other hand, thioglycollate-elicited peritoneal neutrophils were used for phagocytosis and Candida inhibition assay. In some experiments, macrophages were stimulated with Pam 3 CSK 4 (100 ng ml −1 ), Curdlan (100 μg ml −1 ), zymosan (100 μg ml −1 ) or heat-killed C. albicans (HKCA; 5 × 10 6 ml −1 ). Antibodies, reagents and major machines for analyses Antibodies against CD11b (clone: M1/70), F4/80 (BM8), TLR4 (MTS510), TLR2 (T2.5), CXCR2 (TG11), CD4 (GK1.5), CD3 (17A2), CD11c (N418) and β-actin were purchased from BioLegend and used at a 1/200 dilution. Antibodies against CD8 (53–6.7), Ly6G (1A8) and B220 (RA3-6B2) were from BD Bioscience (1/200 dilution). Dectin-1 (2A11) and dectin-2 (D2.11E4) antibodies were from AbD Serotec (1/100 dilution). IκB (L35A5), phosphorylated IκB (14D4), p62 (5114S), K63-ubiquitin (5621S) and LC3A/B (4108S; 1/1,000 dilution for western blotting) antibodies were purchased from Cell Signaling Technology. LC3 (ab51520; 1/200 dilution for immunofluorescence), IKKγ (ab7890; 1/1,000 dilution for western blotting) antibodies were purchased from Abcam. Antibody against His (HIS.H8; 1/200 dilution) was purchased from Thermo Scientific. V5 antibody (PAB11383; 1/5,000 dilution) and HA antibody (HA-7; 1/1,000 dilution) were purchased from Abnova and Sigma, respectively. A20 monoclonal antibody (A-12; 1/50 dilution for immunoprecipitation and western blotting) and IKKγ antibody (FL-419; 2 μg for 200 μg proteins, for immunoprecipitation), NFκB p65 polyclonal antibody (sc-109; 1/50 dilution), 3-MA, rapamycin and NFκB inhibitor (QNZ) were purchased from Santa Cruz. Recombinant CXCL1 was purchased from BioLegend. Pam 3 CSK 4 and curdlan were purchased from Invivogen. Zymosan was purchased from MP Biomedicals. FACS-sorting with MoFlo Legacy (Beckman Coulter) was used for some experiments. Sorted cell populations we used were confirmed to be >95% of purity. FACS Canto II (BD) was used for flow cytometry. Mastercycler realplex [2] and Mastercycler proS (Eppendorf) were used for real-time PCR and conventional PCR, respectively. Zeiss 710 confocal microscopy and the Zeiss Efficient Navigation (ZEN; Carl Zeiss) softwares were used for data acquisition and analysis, respectively. The Fiji software ( http://fiji.sc/Fiji ) was used to determine the intensity of fluorescence. Candida infection, evaluating fungal burdens and histology Sex-matched mice of age 6–8 weeks were infected by intravenous ( i.v. ) injection of C. albicans (ATCC 18804). In some experiments, the same strain of Candida (5 × 10 6 spores per mouse) was intraperitoneally injected. Body weights and survival of mice were evaluated every 24 h until whichever comes first either 18 days post infection or reaching at the human end point approved by the mouse protocol. To measure in vivo fungal burdens, tissue lysates from kidneys and spleens (or fluids from peritoneal lavage) were first treated with H 2 O to lyse host cells (but C. albicans is not lysed by water), and then plated on YPD agar plates and incubated overnight to determine Candida colony-forming units (CFUs). For histological analysis, tissues were harvested 3 days after Candida infection (10 6 i.v. ) and submitted for haematoxylin and eosine and silver staining. Evaluating Candida uptake and intracellular germination Macrophages and neutrophils were stained with antibodies against CD11b, F4/80 (for macrophages) or Ly6G (for neutrophils), and cocultured with same number of Alexa Fluor 647 (AF647)-labelled C. albicans (host cell versus Candida spore numbers as the 1:1 ratio). Cells were fixed with 2% (wt/vol) paraformaldehyde and submitted for flow cytometry. Proportions of AF647-positive host cells were evaluated for macrophages (CD11b + F4/80 + ) and neutrophils (CD11b + Ly6G + ). Since this method also picks up host cells simply attaching to Candida without phagocytosis, we also evaluated cells by confocal microscopy and eye-counted the cells that completely engulfed Candida . As expected, percentages of AF647-positive cells were larger than those of Candida -engulfed cells evaluated by eye-counting; however, the differences in the percentages were proportional and flow cytometry analysis could be used as a substitute to evaluate phagocytosis between groups used in this study. To evaluate Candida germination, coculture of Candida and host cells were set up as described above for the uptake analysis, except that cells were cultured and fixed directly on cover glasses for confocal microscopic analysis. To evaluate host cell death, the live/dead Fixable Violet Dead Cell Stain Kit (Life technologies) was used and dead cells were enumerated with flow cytometry. Evaluating inhibition of Candida expansion Macrophages (BMDMs, thioglycollate-elicited macrophages, splenic CD11b + macrophages and peritoneal F4/80 hi macrophages) and thioglycollate-elicited neutrophils were used for the analyses. To evaluate host cells to inhibit Candida expansion, live Candida was cocultured with host cells at the 1:10 (conidia:host) ratio (termed ‘test samples’). Negative control culture had Candida alone. Twelve hours after coculture, host cells were lysed with water and Candida CFU was determined with YPD plates. Results were obtained with the following formula: Candida Expansion (fold)=[CFU at 12 h]/[CFU at 0 h]; inhibition of Candida expansion (%)=(1−[CFU of test samples at 12 h]/[CFU of negative control at 12 h]) × 100. Evaluation of NFκB activity NFκB activity was evaluated by either one or combination of the following methods. First RAW-Blue cell line (Invivogen), harbouring an NFκB reporter to express SEAP, was used with QUANTI-Blue (Invivogen) to detect SEAP activity with a plate reader (TECAN), as indicated by the manufacturer. RAW-Blue cells express PRRs, such as TLRs and dectin-1. Second, functional NFκB activity was carried out by evaluating the binding of p65 to a target DNA fragment with the NFκB p65 Transcription Factor Assay kit (Thermo scientific). Third, nuclear translocation of NFκB p65 was evaluated by confocal microscopy. Fourth, biochemical analyses to detect phosphorylation of IκB and reduction of total IκB were also carried out by immunoblotting detection. Neutrophil chemotaxis assay Neutrophils were FACS-sorted from the BM of naive mice as CD11b + Ly6G + . Neutrophils (5 × 10 5 ) were plated in the upper chamber of transwell (3-μm pore size; Corning), and CXCL1 was added in the lower chamber. After 1 h of incubation at 37 °C, numbers of migrated cells were determined. Proportion of migrated cells was calculated as follows: chemotaxis (%)={[cell number in the lower chamber with CXCL1]−[cell number in the lower chamber without CXCL1]/(5 × 10 5 )} × 100. Quantitative PCR analysis mRNA expression levels were determined with real-time PCR using the ΔΔ C t method with the KAPA SYBR fast qPCR Master Mix (KAPA Biosystems) and the following primer sets: Cxcl1 (forward: 5′- TGGGATTCACCTCAAGAACA -3′, reverse: 5′- TTTCTGAACCAAGGGAGCTT -3′), Cxcl2 (forward: 5′- CCACCAACCACCAGGCTAC -3′, reverse: 5′- GCTTCAGGGTCAAGGGCAAA -3′), Ccl3 (forward: 5′- ACTGCCTGCTGCTTCTCCTACA -3′, reverse: 5′- AGGAAAATGACACCTGGCTGG -3′), Ccl4 (forward: 5′- AAACCTAACCCCGAGCAACA -3′, reverse: 5′- CCATTGGTGCTGAGAACCCT-3′ ), Tnfaip3 (forward: 5′- TTTGCTACGACACTCGGAAC -3′, reverse: 5′- TTCTGAGGATGTTGCTGAGG -3′), Atg7 (forward: CAGGACAGAGACCATCAGCTCCAC, reverse: TGGCTGCTACTTCTGCAATGATGT ) and Actb (forward: 5′- TGTTACCAACTGGGACGACA -3′, reverse: 5′- CTGGGTCATCTTTTCACGGT -3′). Actb expression was used as an internal control. Results shown are representatives from multiple independent experiments with similar results. Error bars calculated were based on the calculation of RQ-Min=2 − (ΔΔ C t+ T × s.d. (Δ C t)) and RQ-Max=2 − (ΔΔ C t −T × s.d. (Δ C t)) from triplicate wells as suggested by a manufacturer of PCR machines (Applied Biosystems). T × s.d. (Δ C t) is a square root of x 2 + y 2 , where x and y are standard deviations of C t values for a gene of interest and an internal control (β-actin in our case), respectively. Error bars we had indicate RQ-MIN and RQ-MAX, which constitute the acceptable error for a 95% confidence limit according to Student’s t -test. Western blotting and immunoprecipitation Cells were stimulated with Pam 3 CSK 4 (100 ng ml −1 ) or zymosan (100 μg ml −1 ) and lysed with RIPA buffer and NP-40 (for immunoprecipitation) containing protease inhibitor cocktail (P8340, Sigma). Phosphatase inhibitor cocktail II was added for p-IκB detection. To examine the association between A20 and p62, NIH-3T3 cells were co-transfected with expression vectors for A20 and p62 (pcDNA5-A20-V5/His and pMI-p62-HA, respectively) by using Lipofectamine LTX (Invitrogen), as recommended by the supplier. The expression vectors for A20 and p62 were made in our laboratory, as fusions of the V5/His tag in the pcDNA5 backbone (Invitrogen) and the HA tag in the pMX backbone (Cosmobio), respectively. Immunoprecipitation was carried out by using Dynabeads Protein G Immunoprecipitation system (Invitrogen) with specific antibodies, followed by immunoblotting with indicated antibodies as recommended by the supplier. Signal intensity of blotting was determined by densitometry using the NIH-Image J software ( http://rsbweb.nih.gov/ij/ ). Full blot data are shown in Supplementary Fig. 18 . Cell staining for confocal microscopy analyses Cells were cultured on covered glasses. For staining, cells were washed with TBS containing 0.05% (vol/vol) Tween (TBS-T) and permeabilized with 0.25% (vol/vol) Triton in TBS, and then incubated with a primary antibody at 4 °C overnight, followed by staining with secondary antibody conjugated with fluorophore. Cells on cover glass were embedded to slide glass with mounting medium including 4',6-diamidino-2-phenylindole (Prolong Gold, Invitrogen), and analysed for confocal microscopy. The Fiji software ( http://fiji.sc/Fiji ) was used to determine the intensity of fluorescence. Statistical analysis The two-tailed Student’s t -test was used for statistical analyses of two-group comparisons. Multigroup comparisons were performed by a one-way analysis of variance followed by Tukey–Kramer multiple comparisons test. How to cite this article : Kanayama, M. et al . Autophagy enhances NFκB activity in specific tissue macrophages by sequestering A20 to boost antifungal immunity. Nat. Commun. 6:5779 doi: 10.1038/ncomms6779 (2015).